Wide bandgap tunability in complex transition metal oxides by site-specific substitution Fabricating complex transition metal oxides with a tunable bandgap without compromising their intriguing physical properties is a longstanding challenge. Here we examine the layered ferroelectric bismuth titanate and demonstrate that, by site-specific substitution with the Mott insulator lanthanum cobaltite, its bandgap can be narrowed by as much as 1 eV, while remaining strongly ferroelectric. We find that when a specific site in the host material is preferentially substituted, a split-off state responsible for the bandgap reduction is created just below the conduction band of bismuth titanate. This provides a route for controlling the bandgap in complex oxides for use in emerging oxide optoelectronic and energy applications. Bandgap tuning is at the core of current materials research and optoelectronic device applications. Through successful tuning of the bandgap in semiconductors, bandgap–tailored heterostructures including two-dimensional electron gas and tunnelling structures can be realized. Such advancements offer a greater understanding of physics regarding quantum electrodynamics and stimulated emergence of many related devices [1] . Moreover, the ability to tune the bandgap is becoming increasingly important for developing highly efficient solar cells and transparent conducting oxides. For conventional III–V and II–VI semiconductors, simple bandgap tuning has been extremely successful, leading to realization of the structures mentioned above. For example, GaAs has a bandgap of 1.42 eV, which can be continuously tuned down to 0.35 eV or up to 2.12 eV by substituting In or Al for Ga, respectively. Such simple alloying results in a bandgap spectrum of larger than 1 eV. On the other hand, recent breakthroughs in complex oxides have provided an opportunity to incorporate our understanding of semiconductors into the exotic physics of transition metal oxides (TMOs) [2] , [3] . For example, the observation of quantum transport behaviours in several complex oxides manifest a substantial improvement of oxides in terms of their quality, leading to properties that were thought to be unique to semiconductors [4] , [5] . However, substantial and controllable bandgap tuning has yet to be achieved in TMOs, despite intense effort. To tune the bandgap of TMOs, one might consider modifying or substituting the transition metal with another element, because the rigid nature of the bandgap originates mostly from the strongly localized character of the d -electrons. However, what has been observed is that the fascinating physical properties of TMOs arising from the d -electrons disappear with the modified bandgap. Such difficulties have hampered the recent searches for more efficient transparent conducting oxides and low-bandgap photovoltaic oxides [6] , [7] , [8] , [9] , [10] , [11] . Ferroelectric oxides in particular are attracting renewed attention owing to their inherent built-in potential arising from the spontaneous polarization, which could be used to efficiently separate photon-induced electron-hole pairs [7] , [8] , [9] , [10] , [11] . To identify a useful route for effectively controlling the bandgap in complex oxides, we focused on the ferroelectric Bi 4 Ti 3 O 12 (BiT), which has an optical bandgap energy reported between 3.1 and 3.6 eV [12] , [13] , [14] . Unlike typical ferroelectric perovskites such as BaTiO 3 , Pb(Zr,Ti)O 3 or BiFeO 3 , BiT has an Aurivillius phase with a highly anisotropic monoclinic (pseudo-orthorhombic, a =5.450 Å, b =5.406 Å and c =32.832 Å) [15] layered structure with two alternating atomic arrangements; one fluorite-like (Bi 2 O 2 ) 2− layer and two perovskite (Bi 2 Ti 3 O 10 ) 2+ layer blocks connected with an extra oxygen plane, as schematically shown in Fig. 1a . Note that the c axis lattice constant of BiT is about eight times longer than that of usual simple perovskites. The ferroelectric polarization in BiT mainly points along the a axis direction [16] and is known to originate mostly from the perovskite sublayers, i.e., the shift of cations relative to O ions within the perovskite blocks [17] , [18] . One of the most attractive properties of this bismuth-layered material is its excellent sustainability of ferroelectricity even after intrusion of some oxygen vacancies [17] . (Note that simple perovskite-typed ferroelectrics are usually less tolerant to oxygen vacancies). Thus, the unique layered structure of BiT provides an opportunity to examine site-specific substitutional alloying for altering the bandgap without losing the ferroelectricity. The alloying material was selected among simple perovskite TMOs with low bandgap and high absorption ( α ) above the bandgap. La TM O 3 was our natural choice for the perovskite, as La doping is well known for stabilizing the ferroelectricity in BiT (refs. 19 , 20 ). Among La TM O 3 , LaCoO 3 (LCO) is chosen as the alloying material. LCO is a Mott insulator with a small bandgap of 0.1 eV and also a high α originating from the Co 3 d -electronic states [21] . It also has a rhombohedral structure ( a =5.378 Å) with an in-plane lattice mismatch with BiT <1%, readily allowing coherent incorporation into BiT without destroying the overall layered structure. 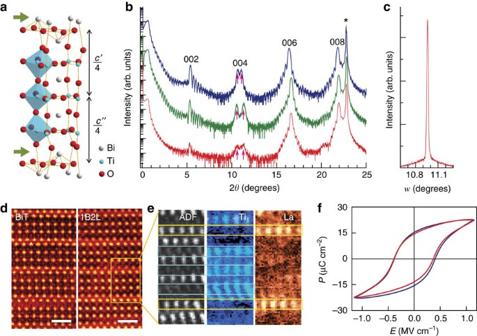Figure 1: Effects of site-specific substitution on structural and ferroelectric properties. (a) Schematic diagram of a half pseudo-orthorhombic unit cell of BiT. The arrows indicate the most probable sites where BiT is substituted by LCO. (b) X-rayθ-2θdiffraction patterns of BiT (blue), 1B1L (green) and 1B2L (red) thin films. The 001 peak from STO substrates and the separation of the 004 peak in BiT–LC are indicated as * and arrows, respectively. (c) X-ray rocking curve of the 008 reflection of 1B2L (full width at half maximum=0.025°). (d) Atomic resolution Z-contrast STEM images are shown for BiT and 1B2L. The overall layered structure of BiT is well preserved despite the incorporation of LC, indicating that some portions of BiT are substituted by La and Co without deteriorating the layered structure. The scale bars correspond to 1 nm. (e) Annular dark field image (ADF) and corresponding elemental maps for Ti and La visualized by EELS from a 1B2L sample. La elemental map shows that La mostly substitutes for Bi in the upper layer of the Bi2O2layer. (f)P(E) hysteresis loops of BiT (blue) and BiT–LC (red). Figure 1: Effects of site-specific substitution on structural and ferroelectric properties. ( a ) Schematic diagram of a half pseudo-orthorhombic unit cell of BiT. The arrows indicate the most probable sites where BiT is substituted by LCO. ( b ) X-ray θ -2 θ diffraction patterns of BiT (blue), 1B1L (green) and 1B2L (red) thin films. The 001 peak from STO substrates and the separation of the 004 peak in BiT–LC are indicated as * and arrows, respectively. ( c ) X-ray rocking curve of the 008 reflection of 1B2L (full width at half maximum=0.025°). ( d ) Atomic resolution Z-contrast STEM images are shown for BiT and 1B2L. The overall layered structure of BiT is well preserved despite the incorporation of LC, indicating that some portions of BiT are substituted by La and Co without deteriorating the layered structure. The scale bars correspond to 1 nm. ( e ) Annular dark field image (ADF) and corresponding elemental maps for Ti and La visualized by EELS from a 1B2L sample. La elemental map shows that La mostly substitutes for Bi in the upper layer of the Bi 2 O 2 layer. ( f ) P ( E ) hysteresis loops of BiT (blue) and BiT–LC (red). Full size image In this article we present a combined experimental and theoretical study on LCO-alloyed BiT (BiT–LC) to elucidate the possiblity of bandgap tuning in complex TMOs. Through site-specific substitutional alloying, we successfully reduce the bandgap as much as ~1 eV, without deterioration of the ferroelectricity of BiT. Moreover, we observe enhanced photoresponses from the alloyed BiT thin films, clearly confirming the bandgap reduction. Thin film samples We used pulsed laser epitaxy (PLE, also known as pulsed laser deposition) to fabricate high quality BiT–LC epitaxial thin films on SrTiO 3 (STO) substrates. Details on the film growth and other experimental setups are given in the Methods section. The fabricated BiT–LC samples were intended to have either one or two pseudo-cubic unit cell layers of LCO incorporated into one unit cell layer of BiT, which hereafter will be nominally called as 1Bi 4 Ti 3 O 12 –1LaCoO 3 (1B1L) or 1Bi 4 Ti 3 O 12 –2LaCoO 3 (1B2L), respectively. (However, in reality, much less Co was incorporated in the films relative to the La substitution as discussed later.) For higher concentrations of LCO alloying, coherent incorporation was not obtained, resulting in a severe degradation of the unique layered structure of BiT. Site-specific substitution The crystal structure of the BiT–LC thin films were characterized using X-ray diffraction (XRD) and Z-contrast scanning transmission electron microscopy (STEM), showing clear evidence of substitutional alloying. Figures 1b and c show XRD θ -2 θ and rocking curve scans, respectively, from BiT–LC thin films. The well-defined thickness fringes observed for most of the peaks in θ -2 θ patterns together with very narrow full width at half maxima ( Δw ~0.025°) in rocking curve scans indicate an atomically smooth surface and interface as well as excellent crystallinity of our thin films. (Note that the full width at half maxima in XRD rocking curves in our films reported here is drastically reduced at least by a factor of three as compared with the values from previous epitaxial films [20] .) Overall peak positions of the main peaks remain unchanged for all the samples up to 1B2L, indicating that the overall Aurivillius structure of BiT is well preserved even after the substitution. This suggests that La and Co were successfully incorporated in BiT. Z-contrast STEM investigations confirm this substitutional alloying, where the characteristic stacking of BiT layers is clearly preserved in BiT–LC as shown in Fig. 1d . A more crucial observation obtained from STEM is the signature of site-specific alloying. Figure 1e shows a magnified annular dark field (ADF) image along with the elemental maps of Ti and La obtained by electron energy-loss spectroscopy (EELS) in a 1B2L sample. The ADF image mostly shows bright features at the Bi and La sites with reduced intensity from the Ti sites. The alternating Bi 2 O 2 and Bi 2 Ti 3 O 10 sublayers are clearly seen. The Ti map obtained using the Ti- L edge shows that Ti is localized within the Bi 2 Ti 3 O 10 sublayer only. The La map shows the asymmetric La substitution for Bi with preferential substitution into the upper layer of Bi within the Bi 2 O 2 sublayer. While considerably less Co incorporation in BiT is detected by STEM–EELS, Co is seen to substitute for Ti. The small amount of Co substitution makes it difficult to determine whether it, similar to La, is asymmetrically incorporated in BiT. However, as discussed later, it is suggested that the La and Co substitution in BiT mostly takes place near the Bi 2 O 2 sublayer region, forming a site-specifically alloyed, self-ordered superstructure. The reduced incorporation of Co relative to La in our thin films seems to originate from the energetically unfavourable electronic state of Co and the different adsorption rate of the elements during the deposition. As Co has two primary valence states in oxides (Co 3+ and Co 2+ ), where Co 2+ is generally more stable, Co substitution in either case for Ti 4+ is more difficult as it requires a compensation of the charge difference, while La 3+ could readily substitute for volatile Bi 3+ . Nevertheless, the impact of Co on the bandgap change is amazingly large as discussed later. Moreover, it has been reported that O vacancies readily form in the Aurivillius structure and prefer sites near the Bi 2 O 2 layer, without compromising the ferroelectricity [17] , [22] , [23] . Therefore, further considering the difference in ionic size as well as electronegativity, we presume that Co preferentially substitutes for Ti next to the Bi 2 O 2 layer accompanying O vacancies to compensate valence difference. Site-specific substitution of LCO is further supported by the XRD θ -2 θ patterns in Fig. 1b . In the XRD θ -2 θ patterns, it should be noted that the peak intensity of higher order peaks (006 and 008) stays almost the same with increasing La and Co substitution as the ones from pure BiT, but that of lower order peaks (002 and 004) decreases as shown in Fig. 1b . This indicates that the short period perovskite structure is conserved on alloying, but the long period Bi 2 O 2 sublayer seems to be disturbed. Another important observation is the separation of the 004 peak in all of our samples, as indicated with the arrows in Fig. 1b . While the origin of the peak separation is not yet clear, it suggests that there is a change in the c /4 lattice of BiT. This might originate from the fact that the distance between upper and lower Bi to O within the Bi 2 O 2 layer is slightly different; the difference between the quarter of the c axis lattice constants (c′/4 and c″/4) is 0.03 nm for the pure BiT film, as schematically shown in Figure 1a . The separation of the 004 peak increases when LCO alloying is introduced, where the c/4 lattice constant difference further increases to ~0.06 nm for both 1B1L and 1B2L. The increase of modulation by alloying with LCO accounts for the observation in STEM, where La preferentially substitutes in the upper Bi layer within the Bi 2 O 2 sublayer in BiT. Persistent ferroelectricity To check the effect of the substitution on the ferroelectric properties of BiT–LC films, we have grown (104)-oriented films on STO (111) covered with SrRuO 3 bottom electrodes. (It was rather difficult to characterize the ferroelectric properties from a c axis oriented film as its primary polar axis is lying along the in-plane direction [24] .) The polarization of a (104)-oriented film is tilted by 54.7° from the normal of the film plane. We measured the polarization ( P ) as a function of electric field ( E ) as shown in Figure 1f . Surprisingly, the overall shape of the P ( E ) loop from BiT–LC is almost identical to that from the pure BiT, indicating its persistent ferroelectricity even after the substitution. The remnant polarization is ~15 μC cm −2 for both BiT and BiT–LC, comparable to the previously reported values of 15.9 μC cm −2 from a (104)-oriented La doped BiT film [24] . (Capacitance and dielectric loss measurements are shown in Supplementary Fig. S1 and further confirm the excellent ferroelectric properties of our thin films). This is an important observation as alloying a simple perovskite-type ferroelectric with heterovalent TMs typically introduces extra charges that induce a (semi-)metallic state and severely degrade the ferroelectricity. Therefore, the persistent ferroelectricity in BiT–LC further supports the model of preferential substitution of Bi 2 O 2 sublayers based on STEM and XRD results described above: The Bi 2 Ti 3 O 10 sublayers remain mostly intact to reveal stable ferroelectricity, even after alloying BiT with La and Co. Optical bandgap control The optical conductivity as a function of photon energy ( σ 1 ( ω )) of our BiT–LC films was measured using spectroscopic ellipsometry as shown in Fig. 2a . While the largely undisturbed Bi 2 Ti 3 O 10 perovskite layers preserve the ferroelectricity in BiT–LC, the changes around the Bi 2 O 2 sublayer modify the optical properties substantially. Charge transfer excitations between O 2 p and Ti 3 d states are known to mainly contribute to the above bandgap absorption of pure BiT [13] . Strong optical transitions start at ~3.55 eV for our BiT film, which we define as the bandgap here to compare different thin film samples on an equal footing (see ref. 13 for a detailed discussion of the spectra). For 1B1L and 1B2L, on the other hand, the bandgap decreased drastically to 3.30 and 2.65 eV, respectively. This could be attributed to LCO that has a larger α , compared with that of typical semiconductors as shown in Fig. 2b . 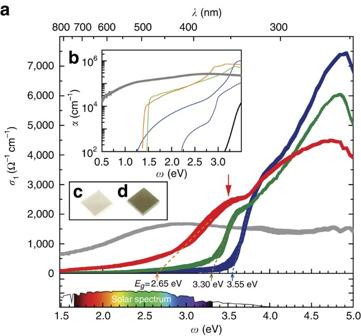Figure 2: Optical property and bandgap change. (a) Optical conductivityσ1(ω) of BiT (blue), 1B1L (green), 1B2L (red) and LCO (grey) show a systematic and substantial decrease in bandgap on site-specific substitution of BiT with La and Co. The thickness of the spectra corresponds to the fitting error bar. Note that the non-zeroσ1(ω) below the bandgap (particularly for 1B2L) may be an artefact, originating from ellipsometry fitting procedure. The extrapolation lines (dashed lines) indicate optical bandgaps (Eg) of ~3.55, ~3.30 and ~2.65 eV for BiT, 1B1L and 1B2L, respectively. The decreased bandgap is mainly due to a state formed below the original bandgap of BiT, as shown by the red arrow. The optical bandgap of 1B2L is green, well within the solar spectrum. (b) Absorption coefficient (α(ω)) of typical semiconductors (GaAs (orange), CdTe (green), crystalline Si (blue) and AlAs (purple)) (data taken from the dielectric constant database of WVASE32 (J.A. Woollam Co.)).α(ω) of STO (black) and LCO (thick grey; measured using ellipsometry) are also shown. LCO has the advantage of a lower bandgap and a higherα(ω) as compared with the typical semiconductors. Photographs of (c) BiT and (d) 1B2L samples intuitively showing the effect of alloying on the bandgap. Figure 2c and d show photographs of BiT and 1B2L on STO, respectively. While BiT is transparent, 1B2L shows a darker colour due to the enhanced absorption of light in the visible wavelength range. The dark colour is not related to unwanted oxygen vacancies typically found in reduced perovskite oxides [25] . In fact, all samples were highly insulating. Moreover, as explained in Supplementary Discussion , our optical spectroscopic analyses preclude the existence of unwanted Co-based phases, and their contribution to the bandgap reduction. Figure 2: Optical property and bandgap change. ( a ) Optical conductivity σ 1 ( ω ) of BiT (blue), 1B1L (green), 1B2L (red) and LCO (grey) show a systematic and substantial decrease in bandgap on site-specific substitution of BiT with La and Co. The thickness of the spectra corresponds to the fitting error bar. Note that the non-zero σ 1 ( ω ) below the bandgap (particularly for 1B2L) may be an artefact, originating from ellipsometry fitting procedure. The extrapolation lines (dashed lines) indicate optical bandgaps ( E g ) of ~3.55, ~3.30 and ~2.65 eV for BiT, 1B1L and 1B2L, respectively. The decreased bandgap is mainly due to a state formed below the original bandgap of BiT, as shown by the red arrow. The optical bandgap of 1B2L is green, well within the solar spectrum. ( b ) Absorption coefficient ( α ( ω )) of typical semiconductors (GaAs (orange), CdTe (green), crystalline Si (blue) and AlAs (purple)) (data taken from the dielectric constant database of WVASE32 (J.A. Woollam Co.)). α ( ω ) of STO (black) and LCO (thick grey; measured using ellipsometry) are also shown. LCO has the advantage of a lower bandgap and a higher α ( ω ) as compared with the typical semiconductors. Photographs of ( c ) BiT and ( d ) 1B2L samples intuitively showing the effect of alloying on the bandgap. Full size image The amount of bandgap change is exceptionally large as compared with the reported values from other doping studies on ferroelectrics. For BiT, the largest bandgap change reported so far was <0.2 eV, referenced to films with a reported gap of 3.64 eV [14] . Other ferroelectrics have similar rigid bandgaps. For example, Pb(Zr,Ti)O 3 shows an experimental bandgap spectrum <0.2 eV by doping [26] , [27] . Thus, we have accomplished wide bandgap tunability (~1 eV), which is about five times greater than what has been reported so far from oxide ferroelectrics. Note that a recent density functional theory work has predicted that substituting the Ti in PbTiO 3 with another metallic element may enhance the polarization while reducing the bandgap [10] . Results from an experimental examination with the exact materials' system, however, have not been reported. Thus, the significantly reduced bandgap experimentally realized in our 1B2L films without reduction of polarization opens up the possibility of discovering new low bandgap ferroelectric materials. It should be noted that the key ingredient to modify the electronic structure of BiT–LC is Co. Although it is present at a smaller concentration than La, the substitution is surprisingly effective in reducing the bandgap. Indeed, doping with only La in BiT is ineffective and known to rather slightly increase the bandgap of BiT (ref. 28 ). This has also been confirmed by testing the substitution with other elements (for example, Ti and Al using LaTiO 3 and LaAlO 3 , respectively) instead of Co. Alloying with these elements did not change the bandgap of BiT at all ( Supplementary Fig. S2 ). Therefore, it is noteworthy to point out that Co has a critical role in manipulating the bandgap of BiT. Electronic structure To understand the evolution of the electronic structure and the effectiveness of Co in reducing the bandgap of BiT–LC, we performed density functional theory calculations. Following the observations from the experiment, we substituted Ti near the Bi 2 O 2 sublayer with Co in our calculation. We focused on Co 2+ in the outer perovskite block in Bi 2 Ti 3 O 10 layer combined with an O vacancy, which we took as the apical O on the outside of the perovskite block consistent with the crystal chemistry of BiT (see Supplementary Methods for details). 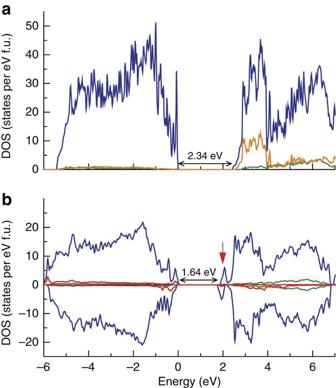Figure 3: Electronic structure. (a) Calculated total electronic density of states (DOS; blue) and projection onto the Bi (green) and Ti (orange) atoms for BiT with Perdew, Burke and Ernzerhof generalized gradient approximation (PBE GGA). The obtained bandgap is 2.34 eV (~1.2 eV smaller than the experimental result as standard density functional theory underestimates the gap value). (b) Calculated total electronic DOS (blue) and projection onto the Bi (green) and Co (red) atoms for the Co:BiT (Bi8Ti5CoO23supercell) with the PBE GGA and the PBE+Umethod withU–J=5 eV for Co atom. Majority and minority spins are shown as positive and negative, respectively. The obtained bandgap for the Co:BiT is 1.64 eV, resulting in ~30% decrease in the bandgap. The theoretical result is in accord with the experimental observation. The origin of the reduced bandgap is additional states below the conduction band of BiT, indicated as a red arrow. This enables charge-transfer excitations below the bandgap of BiT, shown as the same red arrow inFigure 2. Figure 3b shows the calculation result from Co:BiT, in comparison with that for pure BiT in Fig. 3a . As usual, bandgaps are underestimated with standard density functional calculations. The calculated bandgap of 2.34 eV in pure BiT was reduced to 1.64 eV in the Co:BiT supercell, which is comparable to the 30% decrease observed by the ellipsometry. As shown in Fig. 3b , the bandgap reduction in Co:BiT is mainly due to the split-off density of states in the conduction band (indicated as red arrow), meaning that there will be charge-transfer excitations below the pure BiT gap. This is consistent with the additional absorption peak in ellipsometry data, shown as red arrow in Fig. 2 . The split-off states are mainly of Bi 6 p character associated with the Bi atoms nearest to the O vacancy. Therefore, the decreased bandgap in BiT–LC can be attributed to the divalent Co incorporation into the BiT accompanied by O vacancies that pull Bi state down from the conduction band edge. This theoretical result shows that it is possible to obtain the electronic structure in accord with our experimental observations based on Co substitution combined with O vacancies. Such vacancies are to be expected in a Co-substituted material because of the chemistry of Co and, in particular, the fact that the most common oxidation states of Co are +2 and +3. Figure 3: Electronic structure. ( a ) Calculated total electronic density of states (DOS; blue) and projection onto the Bi (green) and Ti (orange) atoms for BiT with Perdew, Burke and Ernzerhof generalized gradient approximation (PBE GGA). The obtained bandgap is 2.34 eV (~1.2 eV smaller than the experimental result as standard density functional theory underestimates the gap value). ( b ) Calculated total electronic DOS (blue) and projection onto the Bi (green) and Co (red) atoms for the Co:BiT (Bi 8 Ti 5 CoO 23 supercell) with the PBE GGA and the PBE+ U method with U – J =5 eV for Co atom. Majority and minority spins are shown as positive and negative, respectively. The obtained bandgap for the Co:BiT is 1.64 eV, resulting in ~30% decrease in the bandgap. The theoretical result is in accord with the experimental observation. The origin of the reduced bandgap is additional states below the conduction band of BiT, indicated as a red arrow. This enables charge-transfer excitations below the bandgap of BiT, shown as the same red arrow in Figure 2 . Full size image Photoelectric response The photocurrent depends on a variety of factors including α , bandgap, carrier mobility and light intensity. To see the effect of reduced bandgap, we measured photocurrent as a function of ω by using a monochromatic light source in the in-plane geometry. As shown in Fig. 4a for 1B2L, the current density as a function of applied electric field J ( E ) for ω smaller than 2.76 eV shows similar curves as dark J ( E ), indicating that there is no absorption of light. Increased photocurrent starts to appear for ω larger than 2.82 eV. 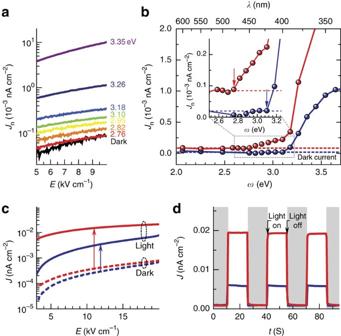Figure 4: Optoelectric properties. (a) Photon energy dependence ofJ(E) of a 1B2L film measured by illuminating light of various wavelength using a monochromator.Jis normalized to the number of photons at each wavelength. (b) Summary of the photoconductance as a function of applied photon energy for BiT (blue) and 1B2L (red) at 10 kV cm−1. Horizontal dashed lines indicate the dark current for each sample. The inset shows magnified version of the dotted squared region. Arrows indicate the onsets of photoconductance at 3.10 and 2.75 eV for BiT and 1B2L, respectively. (c)J(E) curves from BiT (blue) and 1B2L (red) thin films. Illumination of white light by a solar simulator (250 W) enhanced the current level by ~10 and ~35 times for BiT and 1B2L, respectively, indicated by arrows. (d) Photocurrent density recorded from BiT (blue) and 1B2L (red) thin films by switching on and off the solar simulator at 20 kV cm−1. Figure 4b summarizes the wavelength-dependent photoconductance. J for 1B2L starts to increase at 2.82 eV, whereas J for pure BiT does not deviate from dark J until ω reaches 3.18 eV, clearly confirming the enhanced α and photoelectric response due to the reduced bandgap in BiT–LC. Note that the onset values approximately correspond to the bandgap energies shown in Fig. 2 . This means that absorption at these energies below the bandgap of pure BiT yields mobile carriers that can participate in transport, as opposed to absorption that might come from fully localized defect states. Moreover, as there is increased absorption of visible light in BiT–LC owing to the reduced bandgap, one can expect an enhanced total photoelectric response. Figure 4c shows J ( E ) for BiT and 1B2L using a white light with a solar simulator. Both samples show a highly insulating behaviour in the dark. When the sample is illuminated, J increases by approximately an order of magnitude even for pure BiT. A substantially greater enhancement (approximately 35-fold increase of J ) is observed from 1B2L. The enhancement of J in BiT–LC is more obviously shown in Fig. 4d , where the time dependent J shows a clear step-like increase and decrease by turning on and off the light, respectively. This clearly demonstrates the ability of absorbing more photons by the site-specific substitution, which can be in principle converted into electricity. Figure 4: Optoelectric properties. ( a ) Photon energy dependence of J ( E ) of a 1B2L film measured by illuminating light of various wavelength using a monochromator. J is normalized to the number of photons at each wavelength. ( b ) Summary of the photoconductance as a function of applied photon energy for BiT (blue) and 1B2L (red) at 10 kV cm −1 . Horizontal dashed lines indicate the dark current for each sample. The inset shows magnified version of the dotted squared region. Arrows indicate the onsets of photoconductance at 3.10 and 2.75 eV for BiT and 1B2L, respectively. ( c ) J ( E ) curves from BiT (blue) and 1B2L (red) thin films. Illumination of white light by a solar simulator (250 W) enhanced the current level by ~10 and ~35 times for BiT and 1B2L, respectively, indicated by arrows. ( d ) Photocurrent density recorded from BiT (blue) and 1B2L (red) thin films by switching on and off the solar simulator at 20 kV cm −1 . Full size image Site-specific substitution in anisotropic oxides can offer an effective way to tuning bandgaps in complex TMOs. In particular, we showed the example of ferroelectric oxide BiT , where the bandgap could be systematically controlled by site-specific substitutional alloying with LCO. This approach should not be limited to ferroelectrics but could be adapted to other oxide systems that have various exotic and useful characteristics. In addition, while this work has focused on site-specific substitution through the formation of a self-ordered superstructure, we envisage that our finding could be applied to other artificially designed material systems, such as other Aurivillius phase materials, Ruddlesden-Popper series and artificial oxide superlattices [29] , [30] . Thus, our approach may lead to opportunities for more successful integration of intriguing behaviours of complex oxides and other functionalities in electronic and energy applications. Sample fabrication We have fabricated (001)-oriented BiT–LC epitaxial films (~40 nm in thickness) on single crystal (001) STO substrates using PLE with stoichiometric BiT and LCO targets. The thin films were grown with the heater temperature between 700 and 750 °C in 100 mTorr of oxygen. A relatively high laser repetition rate of 10 Hz was used to prevent the loss of volatile Bi in the films. Quarter and half unit cell layers of LCO alternating with quarter unit cell layers of BiT were ablated for growing 1B1L and 1B2L alloys, respectively, by controlling the number of the laser pulses. STEM–EELS Cross-sections of BiT and 1B2L epitaxial films were imaged in a fifth-order aberration corrected Nion UltraSTEM operated at 100 kV. Simultaneous high-angle ADF images and EELS were obtained to investigate the incorporation of La and Co in the BiT matrix. Elemental maps corresponding to the Ti- L 2,3 , Co- L 2,3 and La- M 4,5 edges were produced by subtracting the background using a power law fit and integrating the remaining intensity under each edge in a 30 eV wide window. The acquisition time was 0.1 s per pixel. EELS data are shown in Supplementary Fig. S3 . Ferroelectric characterization To evaluate the ferroelectric polarization, (104)-oriented epitaxial BiT and BiT–LC films were grown on (111) STO substrates covered with SrRuO 3 bottom electrodes using PLE. The polarization in such non- c -axis–oriented thin films is aligned away from the film plane, so that the ferroelectric measurement can readily be performed in capacitor geometry [20] . Pt top electrodes (30-μm diameter) were deposited on the film surfaces using photolithographic lift-off to fabricate capacitors. The PE hysteresis loops were recorded with a standard TF analyzer at 100–500 Hz. Ellipsometry The optical properties of the (001) BiT–LC samples were investigated using a two-modulator generalized ellipsometer [31] , [32] in the wavelength range between 232 and 850 nm (1.46–5.34 eV) at four angles of incidence (55, 60, 65 and 70°). The near-surface region was modelled using a four-medium model: air/surface roughness/film (BiT–LC)/substrate (STO). The surface roughness (typically <5 nm) was modelled using the Bruggeman effective medium approximation [33] consisting of 50% film and 50% voids. (An interface layer was included in some of the calculations, but was not found to improve the fits.) The ellipsometric spectra taken at multiple angles of incidence were then used to determine the spectroscopic dielectric functions ɛ 1 ( ω ) and ɛ 2 ( ω ) of the films, as well as the film thickness. The film thickness was ~40 nm, which was consistent with the values obtained from low-angle X-ray reflection measurements. The data are reported as the optical conductivity σ 1 = ɛ 2 ω/ 4 π . Photoconductance measurements Interdigitated Pt electrodes with a 10-μm separation were patterned using the photolithography lift-off process on (001) BiT–LC films for in-plane photoconductance measurements. The electrodes were then wired using gold wires. Light was illuminated using either a solar simulator (250 W) or a monochromator. For the monochromator, the number of incident photons was determined using a NIST-calibrated photodiode. The current density is then normalized to the number of photons for each wavelength. Density functional calculations We constructed a supercell based on the two formula unit primitive cell of BiT substituting one Ti by Co and removing one O as described in the text to yield a formula Bi 8 Ti 5 CoO 23 . The internal atomic positions were then fully relaxed including the spin polarization, so that Co could carry a moment. The calculation was done within density functional theory using the augmented planewave plus local orbital extension of the general potential linearized augmented planewave method, as implemented in the wien2k code. The initial relaxation was done using the generalized gradient approximation of Perdew, Burke and Ernzerhof with a scalar relativistic approximation. We tested our calculations using the Perdew, Burke and Ernzerhof+ U method with various values of the Coulomb parameter U ; the results were insensitive to U provided that it is large enough to remove the Co d -states from the bandgap. The reason is that the band edge states induced by the substitution come mainly from Bi. How to cite this article: Choi, W. S. et al . Wide bandgap tunability in complex transition metal oxides by site-specific substitution. Nat. Commun. 3:689 doi: 10.1038/ncomms1690 (2012).